The APC/C cofactor Cdh1 prevents replicative stress and p53-dependent cell death in neural progenitors The E3-ubiquitin ligase APC/C-Cdh1 is essential for endoreduplication but its relevance in the mammalian mitotic cell cycle is still unclear. Here we show that genetic ablation of Cdh1 in the developing nervous system results in hypoplastic brain and hydrocephalus. These defects correlate with enhanced levels of Cdh1 substrates and increased entry into the S phase in neural progenitors. However, cell division is prevented in the absence of Cdh1 due to hyperactivation of cyclin-dependent kinases, replicative stress, induction of p53, G2 arrest and apoptotic death of these progenitor cells. Concomitant ablation of p53 rescues apoptosis but not replicative stress, resulting in the presence of damaged neurons throughout the adult brain. These data indicate that the inactivation of Cdh1 in vivo results in replicative stress, cell cycle arrest and cell death, supporting recent therapeutic proposals aimed to inhibit the APC/C in tumours. Proper progression throughout the cell division cycle depends on ubiquitin-dependent degradation of cell cycle regulators at specific stages. Major E3-ubiquitin ligases that target proteins for proteasome-dependent degradation during the cell cycle include the SCF (Skp1/Cullin/F-box) protein complex and the anaphase-promoting complex/cyclosome (APC/C) [1] , [2] , [3] , [4] . The APC/C is responsible for targeting critical regulators for degradation during mitosis and G1 until its activity is inhibited at the G1/S transition. This multimeric complex requires the binding of either Cdc20 or Cdh1, two cofactors that recruit the specific substrates. Cdc20 is essential for the anaphase onset by targeting cyclin B and securin for destruction thus promoting the activation of separase and sister chromatid segregation [3] . Cdh1, on the other hand, replaces Cdc20 during mitotic exit and triggers the ubiquitination of multiple cell cycle regulators (such as aurora kinases, Tpx2, Plk1, A- and B-type cyclins, and so on), thus preventing the accumulation of these proteins during the following G1 phase [3] , [5] . In mammals, genetic ablation of Cdc20 results in metaphase arrest and embryonic lethality at the two-cell stage [6] , [7] . Cdh1 on the other hand is dispensable for the mitotic cell cycle in yeast, Caenorhabditis elegans , Drosophila or mammals (ref. 8 and references herein). During embryonic development, genetic ablation of Cdh1 results in lethality at mid-gestation owing to the requirements for Cdh1 during endoreduplication of trophoblast giant cells [8] , [9] , [10] . This lethal phenotype has prevented the detailed analysis of the effects of complete Cdh1 ablation in postnatal stages although heterozygous mice displayed some susceptibility to mammary gland tumour development in agreement with a tumour-suppressor function for this APC/C cofactor [8] . A specific function of APC/C-Cdh1 in the nervous system was originally proposed after finding high levels of Cdh1 and several core APC/C subunits in postmitotic neurons [11] . In the last few years, several studies have shown that the APC/C can regulate both axonal growth and patterning through Cdh1 (refs 12 , 13 , 14 ), as well as presynaptic axonal differentiation and dendrite morphogenesis by Cdc20 [15] , [16] . Furthermore, APC/C-Cdh1 may play a key role in the organization of synapses [17] , [18] and in homoeostatic plasticity by targeting GluR1 for proteasomal degradation in neurons [19] . Cdh1 heterozygous mice display synaptic and behavioural defects including alterations in neuromuscular coordination and learning [8] , [9] . However, these mice display a normal architecture of the nervous system probably owing to the remaining wild-type Cdh1 allele. The requirements for the APC/C during mitotic exit have been recently used to propose new therapeutic strategies against proliferative diseases such as cancer [20] . Downregulation of APC/C-Cdc20 results in metaphase arrest and subsequent cell death suggesting therapeutic uses for the inhibition of mitotic exit in cancer cells [6] , [21] . One possible complication of these strategies resides in the possible undesired effect of inhibiting APC/C-Cdh1, as lack of Cdh1 activity may result in the accumulation of proliferative molecules such as cyclins or oncogenes such as Pttg1/securin or aurora kinases that could drive increased cellular proliferation. Here, we show that elimination of Cdh1 in the developing nervous system by a Cre recombinase expressed under the nestin regulatory sequences results in defects in the neural progenitor compartment, hydrocephalus (accumulation of cerebrospinal fluid in the cavities of the brain) and death of these mutant mice. This particular requirement for Cdh1 during neurogenesis is related to the ability of Cdh1 to prevent replicative stress in progenitors of the developing brain. In the absence of Cdh1, Sox2- and Sox9-positive neural progenitors display aberrant phosphorylation of H2AX, a marker of replicative stress, and undergo apoptosis. This cell death is prevented after genetic ablation of p53 suggesting that the ubiquitin ligase APC/C-Cdh1 prevents p53-dependent apoptosis as a consequence of replicative stress in the developing cortex. Reduced cortical neurogenesis in Cdh1-null mice Cdh1 is highly expressed in the brain [11] , and we and others previously observed several defects in behavior, neuromuscular coordination and learning, together with abnormal proliferation of progenitor cells in the adult brains of mice with just one functional allele of the Cdh1-encoding gene, known as Fzr1 in mammals [8] , [9] . However, the role of Cdh1 in the murine nervous system has not been studied, as homozygous Fzr1 mutation results in lethality at embryonic day (E)9.5–10.5 owing to an essential role of Cdh1 in the endoreduplication of trophoblast giant cells in the placenta [8] , [9] . We, therefore used Nestin-Cre transgenic mice [22] to eliminate Cdh1 function in the developing nervous system. Fzr1 (Δ/Δ); Nestin-Cre mice were viable but about 50% of them died during the first 2 months of life, whereas Fzr1 (lox/lox) ( n =39) or Fzr1 (+/Δ); Nestin-Cre mice remained viable during that period ( Fig. 1a ). Adult Fzr1 (Δ/Δ); Nestin-Cre mice scored poorly in the object-recognition assay ( Fig. 1b ), suggesting defects in learning that were even stronger than the ones observed in Fzr1 (+/−) heterozygous mice [8] . As both Nestin and Cdh1 are expressed in the mouse retina, we cannot rule out a possible defect in the object-recognition assay owing to the specific ablation of Cdh1 in the eye. Morphological analysis of the skull by computerized axial tomography scan ( Fig. 1c ) showed a progressive increase in the size of Fzr1 (Δ/Δ); Nestin-Cre heads at different stages during postnatal development. This defect was accompanied by the accumulation of liquid in the brain ventricles as detected by nuclear magnetic resonance imaging ( Fig. 1d ). 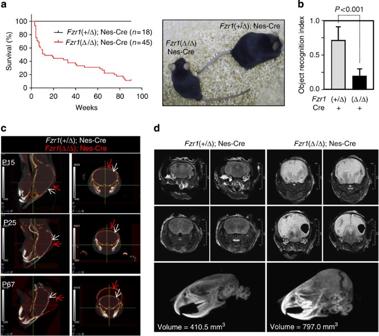Figure 1: Cdh1 depletion in the developing nervous system. (a) Survival curve ofFzr1(Δ/Δ); Nestin-Cre and control mice. A representative picture of 50 week-old littermates is also shown. (b) Results from the object-recognition assay in mutant (Fzr1(Δ/Δ); Nestin-Cre;n=7) and control (Fzr1(+/Δ); Nestin-Cre;n=9) adult (13–25-week-old) mice. Error bars indicate s.e.m. (c) Analysis of the progression of hydrocephalus inFzr1(Δ/Δ); Nestin-Cre mice at P15, P25 and P67 by computerized axial tomography scanning. Figures show an overlap of the cranial shape from mutant (red) or control (white) mice in sagittal (left panels) or coronal (right panels) sections. (d) Coronal T2-weighted magnetic resonance images of 9-week-oldFzr1(Δ/Δ); Nestin-Cre and control brains (top panels). Whereas control ventricles are barely visible (arrow),Fzr1(Δ/Δ); Nestin-Cre brains display a marked enlargement of the ventricles with a noticeable presence of liquid all over the brain (shown by the whitish aspect of the cortex). Figure 1: Cdh1 depletion in the developing nervous system. ( a ) Survival curve of Fzr1 (Δ/Δ); Nestin-Cre and control mice. A representative picture of 50 week-old littermates is also shown. ( b ) Results from the object-recognition assay in mutant ( Fzr1 (Δ/Δ); Nestin-Cre; n =7) and control ( Fzr1 (+/Δ); Nestin-Cre; n =9) adult (13–25-week-old) mice. Error bars indicate s.e.m. ( c ) Analysis of the progression of hydrocephalus in Fzr1 (Δ/Δ); Nestin-Cre mice at P15, P25 and P67 by computerized axial tomography scanning. Figures show an overlap of the cranial shape from mutant (red) or control (white) mice in sagittal (left panels) or coronal (right panels) sections. ( d ) Coronal T2-weighted magnetic resonance images of 9-week-old Fzr1 (Δ/Δ); Nestin-Cre and control brains (top panels). Whereas control ventricles are barely visible (arrow), Fzr1 (Δ/Δ); Nestin-Cre brains display a marked enlargement of the ventricles with a noticeable presence of liquid all over the brain (shown by the whitish aspect of the cortex). Full size image In agreement with the in vivo imaging data, brains of young (P10–P35) Fzr1 (Δ/Δ); Nestin-Cre mice displayed enlarged ventricles, accompanied by thinned cortex and agenesis of the corpus callosum ( Fig. 2a and Supplementary Fig. S1 ). Closer inspection of coronal brain sections from P10 Cdh1-deficient mice in conventional hematoxylin and eosin stainings revealed a significant reduction (26.6±1.6%; mean reduction±s.e.m. ; n =3; Student’s t -test P <0.01) in the thickness of the cortex and the absence of the corpus callosum ( Fig. 2a ). The thinning in the postnatal cortex correlated with a decrease in the thickness of the cortical plate at E14.5, revealed by antibodies against Tbr1, a marker for postmitotic neurons, along with an increase in the area occupied by Tbr2-positive intermediate progenitor cells ( Fig. 2b ). Cdh1 is actually highly expressed in embryonic brains with strong representation in the subventricular area ( Supplementary Fig. S2 ). Quantitation indeed showed that the number of Tbr2+ progenitor cells was increased, whereas the number of Tbr1+ neurons was decreased in mutant cortices relative to wild types ( Fig. 2b ), suggesting that Cdh1 is required for the timely production of cortical neurons. We also scored reduced numbers of bromodeoxyuridine (BrdU)-retaining cells, corresponding to postmitotic neurons, in the cortex of P10 Fzr1 (Δ/Δ); Nes-Cre mice born from females injected with BrdU at gestational day E15.5, a developmental time point in which layer II/III cortico-cortical callosal pyramidal neurons are being generated from cortical progenitors. Cdh1-deficient brains showed a significant reduction in the number of neurons generated in that assay ( Fig. 2c ), indicating that neurogenesis was severely affected when Cdh1 is deleted in Nestin+ cortical progenitors. Immunofluorescence for Satb2, a postmitotic marker for upper-layer neurons in the neocortex, and Ctip2, a marker preferentially expressed in layer V neurons revealed that the reduction was even more evident in the deep layers (V–VI) of the mutant cortex ( Fig. 2d ). 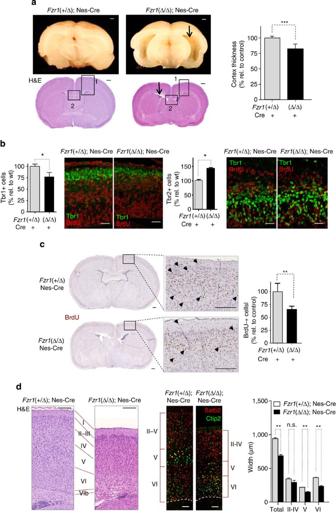Figure 2: Cdh1 ablation results in defective neurogenesis. (a) Macroscopic (P21) and microscopic (P10) brain sections ofFzr1(Δ/Δ); Nestin-Cre and control mice. Cdh1-deficient brains display enlarged ventricles (arrows) and reduced thickness in the cortex. Cortex thickness is quantified in P10 Cdh1-null and control newborns (n=6 per genotype). (b) Tbr1, Tbr2 and BrdU immunofluorescence in E14.5 cortices. Histograms show the quantification of Tbr1 and Tbr2 positive cells. (c) Reduced generation of neurons in Cdh1-deficient brains. Detection of BrdU-retaining positive cells in P10 sections after injection of BrdU in E15.5 embryos. (d) Detailed micrographs of area 1 (area 2 is detailed inSupplementary Fig. S1) from panel (a) indicating the different layers of the cortex (left panels). Immunofluorescence for Satb2 (red) and Ctip2 (green; middle panels). Thickness of layers II–VI is quantified in the histogram based on these markers. (a–d) are coronal sections. (b–d),n=3 per genotype. *P<0.05; **P<0.01; ***P<0.001; n.s.=not significant; Student’st-test. Error bars indicate s.e.m. Scale bar, 500 μm (a), 25 μm (b), 250 μm (cand black bars ind) and 75 μm (d, white bars). Figure 2: Cdh1 ablation results in defective neurogenesis. ( a ) Macroscopic (P21) and microscopic (P10) brain sections of Fzr1 (Δ/Δ); Nestin-Cre and control mice. Cdh1-deficient brains display enlarged ventricles (arrows) and reduced thickness in the cortex. Cortex thickness is quantified in P10 Cdh1-null and control newborns ( n =6 per genotype). ( b ) Tbr1, Tbr2 and BrdU immunofluorescence in E14.5 cortices. Histograms show the quantification of Tbr1 and Tbr2 positive cells. ( c ) Reduced generation of neurons in Cdh1-deficient brains. Detection of BrdU-retaining positive cells in P10 sections after injection of BrdU in E15.5 embryos. ( d ) Detailed micrographs of area 1 (area 2 is detailed in Supplementary Fig. S1 ) from panel ( a ) indicating the different layers of the cortex (left panels). Immunofluorescence for Satb2 (red) and Ctip2 (green; middle panels). Thickness of layers II–VI is quantified in the histogram based on these markers. ( a – d ) are coronal sections. ( b – d ), n =3 per genotype. * P <0.05; ** P <0.01; *** P <0.001; n.s.=not significant; Student’s t -test. Error bars indicate s.e.m. Scale bar, 500 μm ( a ), 25 μm ( b ), 250 μm ( c and black bars in d ) and 75 μm ( d , white bars). Full size image The robust expression of Cdh1 in postmitotic neurons [11] and its reported function in the control of axon growth and patterning in the developing mammalian brain [12] suggested the possibility that corpus callosum agenesis and cortical reduced thickness were also the result of a failure of differentiating neurons to extend their axons. Interestingly, we examined the cellular density in cortical layer VI in P10 Cdh1-null mice and found a significant increase (4,268±89 s.e.m. cells mm −2 in Cdh1-null versus 3,274±78 cells mm −2 in wild-type brains; n =3; Student’s t -test P <0.01), which could be because of the defect in establishing normal projections by Cdh1-deficient neurons. This was consistent with an evident reduction in the number of cortical axonal projections in immunohistochemical stainings for myelin basic protein, a marker of axon myelin sheath ( Supplementary Fig. S1 ). These data suggest that both reduced neurogenesis and defective axonal projections may contribute to reduced cortical thickness in the absence of Cdh1. However, other major forebrain axon tracts such as the anterior and hippocampal commissures appeared normal, suggesting that the defect in callosal development did not result from global defects in axon growth or midline development. Generation of a conditional Cdh1 mutant from a Sox2 promoter also resulted in reduced size, problems in motility, coordination by P10 and increased perinatal death. These defects were accompanied by a similar cortical phenotype as well as increased apoptosis in multiple tissues ( Supplementary Fig. S3 ). All these data together indicated that Cdh1 might be essentially required for cortical neurogenesis during fetal development. Lack of Cdh1 results in abnormal DNA replication To elucidate the possible cause of these defects, we analysed cell proliferation during embryonic development in these mutant mice. By E14.5, many known Cdh1 substrates implicated in mitotic progression, including aurora A, aurora B, Tpx2 or Cyclin B1 were upregulated in Cdh1-deficient embryos ( Fig. 3a,b and Supplementary Fig. S4 ). Accordingly, whereas the labelling for proliferation marker Ki67 was restricted to the ventricular germinal layer in E14.5 wild-type embryos, it was more extended in Cdh1-null brains ( Fig. 3c ). Moreover, E14.5 mutant embryos displayed an increased incorporation of the nucleotide analogue BrdU, suggesting increased DNA replication in vivo ( Fig. 3d ). 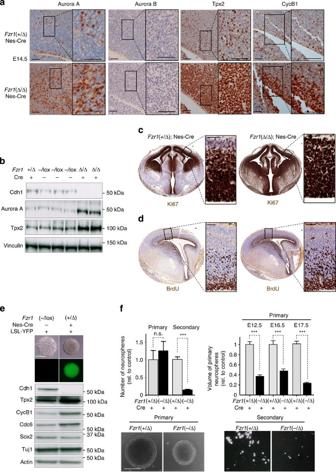Figure 3: Upregulation of Cdh1 substrates and increased proliferation in Cdh1-deficient neural progenitors. (a) Protein level of several Cdh1 substrates in histological sections of E14.5 brains detected by immunohistochemistry with specific antibodies against the indicated proteins (brown signal). The quantification of these data is shown asSupplementary Material. (b) Levels of Cdh1 substrates in E15.5 brain lysates from the indicated genotypes. Vinculin was used as a loading control. (c) Increase in the proliferation marker Ki67 in E14.5Fzr1(Δ/Δ); Nestin-Cre brains compared with controls. (d) Increased BrdU incorporation in E14.5Fzr1(Δ/Δ); Nestin-Cre brains compared with controls 6 h after the injection of BrdU (100 μg BrdU g−1) in the pregnant female. (e) Analysis of Nestin-Cre expression and activity using the Rosa26-LSL-YFP reporter allele in cultured neurospheres. Cre activity results in the excision of the LSL cassette and expression of YFP. This activity also results in the genetic ablation of Cdh1 and the stabilization of several Cdh1 substrates such as Tpx2, Cyclin B1, geminin or Cdc6 in mutant neurospheres. Actin is used as a protein loading control, whereas the presence of Sox2 and Tuj1 indicate a mixture between progenitors and neurons in these neurospheres. (f) Quantification of the number and size of primary or secondary neurospheres generated from E14.5 (left histograms) or E12.5–17.5 (right histograms) embryonic brains. (n=3 embryos per genotype). ***P<0.001; n.s.=not significant; Student’st-test. Error bars indicate s.e.m. (a) and (d) are sagital sections; (c) are coronal sections. Scale bar, 50 μm (a,c,d) or 100 μm (f). Figure 3: Upregulation of Cdh1 substrates and increased proliferation in Cdh1-deficient neural progenitors. ( a ) Protein level of several Cdh1 substrates in histological sections of E14.5 brains detected by immunohistochemistry with specific antibodies against the indicated proteins (brown signal). The quantification of these data is shown as Supplementary Material . ( b ) Levels of Cdh1 substrates in E15.5 brain lysates from the indicated genotypes. Vinculin was used as a loading control. ( c ) Increase in the proliferation marker Ki67 in E14.5 Fzr1 (Δ/Δ); Nestin-Cre brains compared with controls. ( d ) Increased BrdU incorporation in E14.5 Fzr1 (Δ/Δ); Nestin-Cre brains compared with controls 6 h after the injection of BrdU (100 μg BrdU g −1 ) in the pregnant female. ( e ) Analysis of Nestin-Cre expression and activity using the Rosa26-LSL-YFP reporter allele in cultured neurospheres. Cre activity results in the excision of the LSL cassette and expression of YFP. This activity also results in the genetic ablation of Cdh1 and the stabilization of several Cdh1 substrates such as Tpx2, Cyclin B1, geminin or Cdc6 in mutant neurospheres. Actin is used as a protein loading control, whereas the presence of Sox2 and Tuj1 indicate a mixture between progenitors and neurons in these neurospheres. ( f ) Quantification of the number and size of primary or secondary neurospheres generated from E14.5 (left histograms) or E12.5–17.5 (right histograms) embryonic brains. ( n =3 embryos per genotype). *** P <0.001; n.s.=not significant; Student’s t -test. Error bars indicate s.e.m. ( a ) and ( d ) are sagital sections; ( c ) are coronal sections. Scale bar, 50 μm ( a , c , d ) or 100 μm ( f ). Full size image We next decided to further analyse the proliferative behavior of neural progenitors by generating neurospheres in culture. We first tested whether Nestin-Cre was active in these neurospheres by introducing in these animals a Rosa26-lox-STOP-lox(LSL)-YFP allele ( Fig. 3e ). The activity of Cre recombinase on this allele results in the excision of the LSL cassette, thus driving the expression of the yellow fluorescent protein (YFP) from the ubiquitously expressed Rosa26 locus. Cdh1 is normally expressed in these primary neurospheres and its ablation resulted in the overexpression of its known substrates such as Tpx2, Cyclin B1, Geminin or Cdc6 ( Fig. 3e ) as well as the reduction in cell cycle inhibitors such as p21 Cip1 or p27 Kip1 , a possible consequence of the increased levels of the Cdh1-target Skp2, an F-box protein that targets these cell-cycle inhibitors for degradation ( Supplementary Fig. S4 ). Genetic elimination of Cdh1 did not alter the number of primary neurospheres obtained from E14.5 cortices, but incorporation of the nucleotide analogue EdU in 3–4-day cultures of primary neurospheres was augmented in Cdh1-null neurospheres ( Fig. 4a ) in agreement with the increased incorporation of BrdU in utero ( Fig. 3d ). Intriguingly, the size of these primary neurospheres was significantly reduced (20–50% of the control volume; Fig. 3f ) when using E12.5–E17.5 embryos. In agreement with these observations, the number of secondary neurospheres generated after disaggregation of the E14.5 primary neurospheres was markedly reduced ( Fig. 3f ). These results suggested that Cdh1 supports normal proliferation of neural progenitors mostly by regulating their entry into the S phase. 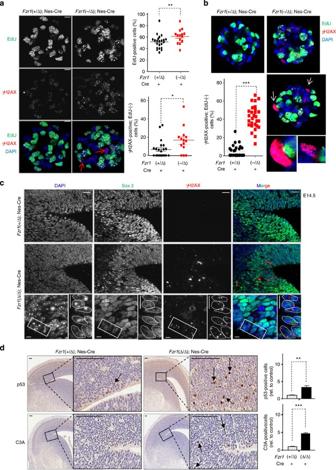Figure 4: Cdh1 ablation results in replicative stress and a DNA-damage-like response in neural progenitors. (a) EdU and γH2AX immunofluorescence in primary neurospheres. Histograms show the quantification of EdU incorporation and γH2AX-positive/EdU-negative cells in these cultures. (b) EdU and γH2AX immunofluorescence in secondary neurospheres and quantification of γH2AX-positive/EdU-negative cells. Cdh1-deficient secondary neurospheres also display strong pan-nuclear γH2AX staining (white arrows). (c) Accumulation of phosphorylated H2AX (γH2AX; red) in neural progenitors (Sox2 staining, green) in the ventricular area of the brain from E14.5 Cdh1-null embryos. 4′,6-diamidino-2-phenylindole (DAPI), DNA. Scale bars, 25 μm (top panels) or 10 μm (bottom panels). (d) Increased p53 and active caspase-3 staining in E14.5 Cdh1-deficient embryo brains. Scale bars, 100 μm. Histograms show the quantification of positive cells for the different markers. *P<0.05; **P<0.01; ***P<0.001; Student’st-test. Error bars indicate s.e.m.n=3 clones per genotype in all these assays. Figure 4: Cdh1 ablation results in replicative stress and a DNA-damage-like response in neural progenitors. ( a ) EdU and γH2AX immunofluorescence in primary neurospheres. Histograms show the quantification of EdU incorporation and γH2AX-positive/EdU-negative cells in these cultures. ( b ) EdU and γH2AX immunofluorescence in secondary neurospheres and quantification of γH2AX-positive/EdU-negative cells. Cdh1-deficient secondary neurospheres also display strong pan-nuclear γH2AX staining (white arrows). ( c ) Accumulation of phosphorylated H2AX (γH2AX; red) in neural progenitors (Sox2 staining, green) in the ventricular area of the brain from E14.5 Cdh1-null embryos. 4′,6-diamidino-2-phenylindole (DAPI), DNA. Scale bars, 25 μm (top panels) or 10 μm (bottom panels). ( d ) Increased p53 and active caspase-3 staining in E14.5 Cdh1-deficient embryo brains. Scale bars, 100 μm. Histograms show the quantification of positive cells for the different markers. * P <0.05; ** P <0.01; *** P <0.001; Student’s t -test. Error bars indicate s.e.m. n =3 clones per genotype in all these assays. Full size image Cdh1 modulates Cdk activity to prevent replicative stress Cdh1-deficient fibroblasts are known to display a shorter G1 phase, early entry into the S phase and signs of senescence [8] , [9] . We therefore asked whether the increased entry into the S phase was causing replicative defects in these neural progenitors. Phosphorylation of H2AX (γH2AX) is normally present at low levels and in a dot pattern during normal replication of cells, but is eliminated as cells exit from the S phase and progress to mitosis. Lack of Cdh1 resulted in the accumulation of γH2AX both in primary and secondary neurospheres ( Fig. 4a,b ). Importantly, this signal was significantly increased in EdU-negative Cdh1-null cells, suggesting the presence of DNA damage beyond the S phase. Cdh1-null secondary neurospheres also presented increased levels of replicative stress, indicated by the presence of strong pan-nuclear γH2AX signals (in 46% of Cdh1-null versus 11% control neurospheres; Fig. 4b ). The aberrant γH2AX signal was present in both Sox9-(as analysed in three different embryos) and Sox2-positive cells of the ventricular layer ( Fig. 4c ), whereas this signal was not observed in control embryos indicating that lack of Cdh1 induced replicative stress in these neural progenitors in vivo . Importantly, replicative stress was accompanied by the induction of p53 and apoptosis ( Fig. 4d ). The cellular response to replicative stress in the absence of Cdh1 increased in a progressive manner during development (E12.5–E16.5; Supplementary Fig. S5 ). Genetic ablation of Cdh1 driven by the Sox2 promoter similarly resulted in replicative stress, induction of p53 and apoptosis ( Supplementary Fig. S6 ). Cdh1 targets for degradation of multiple proteins involved in many different pathways. However, we reasoned that one of the major consequences of lack of Cdh1 is the hyperactivation of Cdks because of the increased levels of cyclins and decreased levels of Cdk inhibitors ( Fig. 3 and Supplementary Fig. S4 ) during G1. We therefore explored the effect of partially inhibiting Cdks in Cdh1-null cells using the small-molecule inhibitor roscovitine. Partial inhibition of Cdks using a low dose of the inhibitor 3 days after seeding the cells prevented the replicative stress observed in Cdh1-deficient cells after disaggregation of secondary neurospheres ( Fig. 5a ). Importantly, this leads to increased proliferation (as scored by EdU incorporation; Fig. 5b ), suggesting that both the replicative stress and the defective proliferation is at least partially induced by increased Cdk activation in the absence of Cdh1. Similar results were found in cells obtained from primary neurospheres ( Supplementary Fig. S7 ), although the effect of roscovitine was not as marked, in agreement with the increased presence of replicative stress in secondary neurospheres ( Fig. 4a,b ). In addition, whereas high concentration of roscovitine inhibited proliferation (a well-known effect), low dose of this inhibitor did not induce proliferation in wild-type cells and actually slightly increased the γH2AX signal ( Supplementary Fig. S7 ), indicating a specific protective effect of roscovitine in Cdh1-null cells. The addition of nucleosides to these cultures also resulted in a partial protective effect in agreement with recent observations on the relevance of nucleotide levels to prevent replicative stress [23] . 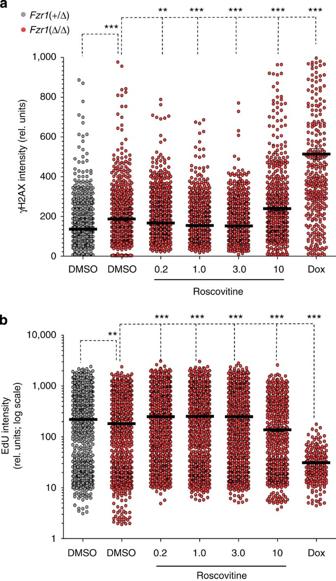Figure 5: Replicative stress in Cdh1-deficient neural progenitors is prevented by partial inhibition of Cdk activity. (a) Quantification of γH2AX intensity in control (grey) or Cdh1-deficient (red) neural progenitors from secondary neurospheres treated for 8 h with the indicated dose of Roscovitine (μM) or Doxorubicin (0.5 μg ml−1) using HTM. (b) Quantification of EdU intensity in control (grey) or Cdh1-deficient (red) neural progenitors from secondary neurospheres treated for 8 h with the indicated dose of Roscovitine (μM) or Doxorubicin (0.5 μg ml−1) using HTM. In the last 30 min of the treatment they were in the presence of EdU (10 μM). Doxorubicin is used as a positive control of DNA damage accumulation (γH2AX staining) and as a negative control of proliferation (absence of EdU incorporation). Data are representative of three independent analyses. **P<0.01; ***P<0.001; Student’st-test. At least 3,000 cells per condition were analysed. Data represent one representative experiment out of three replicates. Figure 5: Replicative stress in Cdh1-deficient neural progenitors is prevented by partial inhibition of Cdk activity. ( a ) Quantification of γH2AX intensity in control (grey) or Cdh1-deficient (red) neural progenitors from secondary neurospheres treated for 8 h with the indicated dose of Roscovitine (μM) or Doxorubicin (0.5 μg ml −1 ) using HTM. ( b ) Quantification of EdU intensity in control (grey) or Cdh1-deficient (red) neural progenitors from secondary neurospheres treated for 8 h with the indicated dose of Roscovitine (μM) or Doxorubicin (0.5 μg ml −1 ) using HTM. In the last 30 min of the treatment they were in the presence of EdU (10 μM). Doxorubicin is used as a positive control of DNA damage accumulation (γH2AX staining) and as a negative control of proliferation (absence of EdU incorporation). Data are representative of three independent analyses. ** P <0.01; *** P <0.001; Student’s t -test. At least 3,000 cells per condition were analysed. Data represent one representative experiment out of three replicates. Full size image A DNA-damage-like response accompanied by G2 arrest To further understand whether the increased entry into the cell cycle in the presence of replicative defects was accompanied not only by death but also by defective cell division, we analysed the pattern of phosphorylation of histone H3 (pH3). This signal shows a spotted pattern during late G2, whereas mitotic cells are characterized by fully condensed chromosomes positive for the pH3 mark [24] . As observed in Fig. 6a , there was a marked increase in the percentage of pH3-positive cells with spotted pattern (G2-like) in the cortex of E14.5 Cdh1-deficient embryos. These cells frequently displayed duplicated centrosomes ( Fig. 6b ) and approximately a twofold increase in nuclear volume ( Fig. 6c ), suggesting a DNA content of 4 N and confirming that these cells were arrested after S phase, a phase in which centrosomes are duplicated. 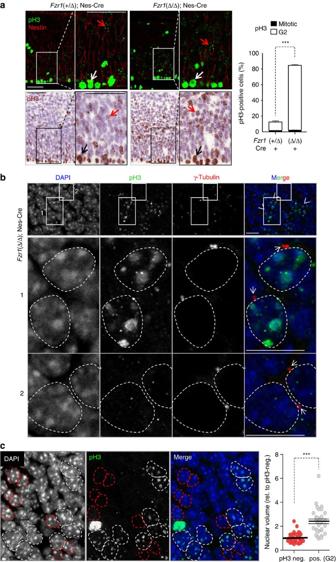Figure 6: Accumulation of G2-like cells in the neuroepithelium of Cdh1-null brains. (a) Staining of phospho-histone H3 (pH3) (red arrows) showing an increase in the number of G2-pattern pH3-positive cells in E14.5 Cdh1-deficient brains. The percentage of G2- (red arrows) or mitotic-pH3-positive (white or black arrows) cells is shown in the histogram. (n>1,000 cells per genotype). (b) The presence of two centrosomes (γ-tubulin red staining; arrowheads) in cells with the spotted pH3 (green) pattern suggests the accumulation of G2 cells in Cdh1-deficient mice (inset 1). As a control only one centrosome is observed in cells negative for pH3 (inset 2). DNA is in blue. Note that centrosomes are not evident in all cells owing to the thickness (5 μm) of the section. (c), Quantification of the nuclear volume of pH3-negative (white lines) and pH3-positive cells (red lines) in the cortex ofFzr1(Δ/Δ);Nes-Cre embryos. The nuclear volume of at least 40 cells per genotype was calculated. In (a) and (c) three diferent embryos per geneotype were analysed. ***P<0.001; Student’st-test. Error bars indicate s.e.m. Scale bar, 10 μm. Figure 6: Accumulation of G2-like cells in the neuroepithelium of Cdh1-null brains. ( a ) Staining of phospho-histone H3 (pH3) (red arrows) showing an increase in the number of G2-pattern pH3-positive cells in E14.5 Cdh1-deficient brains. The percentage of G2- (red arrows) or mitotic-pH3-positive (white or black arrows) cells is shown in the histogram. ( n >1,000 cells per genotype). ( b ) The presence of two centrosomes (γ-tubulin red staining; arrowheads) in cells with the spotted pH3 (green) pattern suggests the accumulation of G2 cells in Cdh1-deficient mice (inset 1). As a control only one centrosome is observed in cells negative for pH3 (inset 2). DNA is in blue. Note that centrosomes are not evident in all cells owing to the thickness (5 μm) of the section. ( c ), Quantification of the nuclear volume of pH3-negative (white lines) and pH3-positive cells (red lines) in the cortex of Fzr1 (Δ/Δ);Nes-Cre embryos. The nuclear volume of at least 40 cells per genotype was calculated. In ( a ) and ( c ) three diferent embryos per geneotype were analysed. *** P <0.001; Student’s t -test. Error bars indicate s.e.m. Scale bar, 10 μm. Full size image As Cdh1 has been reported to modulate axonal growth and patterning [12] , we also tested the differentiation potential of these mutant neural progenitors. Cdh1-null neural progenitors displayed normal ratios of symmetric (leading to two progenitors or two neurons) versus asymmetric (leading to one progenitor+one neuron) cell divisions in vitro ( Fig. 7a,b ), thus indicating that Cdh1 is not required for asymmetric division. Importantly, Cdh1-null cells displayed increased γH2AX signals in these assays ( Fig. 7c ). We also isolated and cultured postmitotic neurons from E14.5 cortices and stained them for β-III-tubulin. A significant number of the neurons generated from Cdh1-null E14.5 brains displayed abnormal morphology, with poorly developed neurites and picnotic nuclei ( Fig. 7d ) in agreement with cell death induced by Cdh1 loss, as reported previously in postmitotic neurons [25] . All together, these data suggest that, in addition to other possible defects in neurite outgrowth, lack of Cdh1 results in an abnormal proliferative response in the developing brain in which neural progenitors display an accelerated entry into the S phase, replicative stress, arrest in a G2-like stage and/or cell death in the presence of p53. 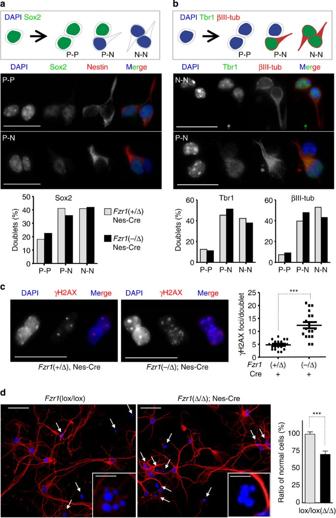Figure 7: Differentiation of Cdh1-null neural progenitors. (a) Immunofluorescence of Sox2 and Nestin in cell doublets originated in differentiation medium. P=progenitor; N=neuron. (b) Similar staining for Tbr1 and βIII-tubulin. P=progenitor; N=neuron. (c) Quantification of DNA damage accumulated in the doublets. (d) Culture of primary cortical neurons from E14.5 embryos. Abnormal cells (arrows and insets) with lack of neurites and possible apoptotic nuclei are indicated by arrows and quantified in the histogram. ***P<0.001; Student’st-test.n=3 clones per genotype. Error bars indicate s.e.m. Data are not significantly different in (a) and (b) (Student'st-test,P>0.05). Scale bar are 25 μm. Scale bars, 50 μm (a), 25 μm (b–d) and 10 μm (insets ind). Figure 7: Differentiation of Cdh1-null neural progenitors. ( a ) Immunofluorescence of Sox2 and Nestin in cell doublets originated in differentiation medium. P=progenitor; N=neuron. ( b ) Similar staining for Tbr1 and βIII-tubulin. P=progenitor; N=neuron. ( c ) Quantification of DNA damage accumulated in the doublets. ( d ) Culture of primary cortical neurons from E14.5 embryos. Abnormal cells (arrows and insets) with lack of neurites and possible apoptotic nuclei are indicated by arrows and quantified in the histogram. *** P <0.001; Student’s t -test. n =3 clones per genotype. Error bars indicate s.e.m. Data are not significantly different in ( a ) and ( b ) (Student's t -test, P >0.05). Scale bar are 25 μm. Scale bars, 50 μm ( a ), 25 μm ( b – d ) and 10 μm (insets in d ). Full size image A cellular response to Cdh1 deficiency in ependymal cells As Fzr1 (Δ/Δ); Nes-Cre mice developed hydrocephalus, we first examined the choroid plexus that showed no gross morphological aberrancies and absence of signs of replicative stress or damage ( Supplementary Fig. S8 ). Next, we tested whether the DNA damage was present in the ependymal layer lining the ventricular system of the brain. These cells are originated from neural progenitors during late embryonic development [26] , and defective integrity of this ependymal layer is known to lead to hydrocephalus [27] , [28] . As shown in Fig. 8 , Cdh1-null ependymal cells displayed defective staining for S100β, a marker of mature ependymal cells, suggesting abnormal maturation and defective control of the cerebrospinal fluid in these mutant ventricles. Importantly, these ependymal cells displayed all the defects described above, including increased expression of Cdh1 substrates (aurora B and Tpx2; n =3 different embryos) Ki67 and PCNA signals (suggesting unscheduled cell cycle entry and increased DNA replication), the γH2AX signal (replicative stress), as well as p53 induction and increased pH3 signal without mitotic figures suggesting G2 arrest ( Fig. 8a,b ). These cell defects were present both during late embryonic development (E18.5) as well as in postnatal stages (P10; Fig. 8 ) in which ependymal cells are normally quiescent [26] . 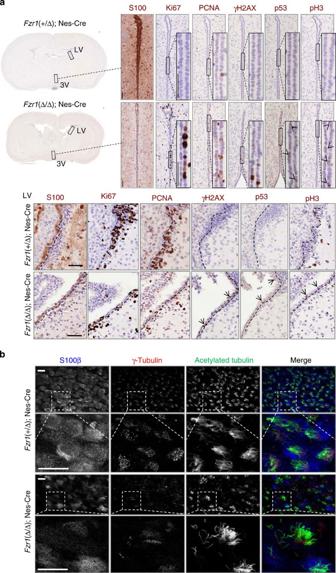Figure 8: Alterations in Cdh1-deficient ependymal cells. (a) Proliferation markers such as Ki67 or PCNA are present in the ependymal layer of mutant but not control mice both in the third ventricle (3V, upper panels) and the lateral ventricles (LV, bottom panels). These markers are accompanied by persistent DNA damage (γH2AX signal), increased p53 levels and phospho-histone H3 (pH3) staining in the absence of mitotic figures suggesting G2 arrest. Some positive cells for these markers are indicated by arrows. On the other hand,Fzr1(Δ/Δ); Nestin-Cre ependymal cells display deficient S100 staining, a marker of mature ependymal cells. Scale bars, 50 μm. (b) Costaining for S100β, acetylated-tubulin and γ-tubulin inen facewhole-mount preparations of the wall of the lateral ventricle of P10 mice confirmed decreased immunoreactivity of S100β and density of multiciliated ependymal cells. Scale bar, 25 μm. Figure 8: Alterations in Cdh1-deficient ependymal cells. ( a ) Proliferation markers such as Ki67 or PCNA are present in the ependymal layer of mutant but not control mice both in the third ventricle (3V, upper panels) and the lateral ventricles (LV, bottom panels). These markers are accompanied by persistent DNA damage (γH2AX signal), increased p53 levels and phospho-histone H3 (pH3) staining in the absence of mitotic figures suggesting G2 arrest. Some positive cells for these markers are indicated by arrows. On the other hand, Fzr1 (Δ/Δ); Nestin-Cre ependymal cells display deficient S100 staining, a marker of mature ependymal cells. Scale bars, 50 μm. ( b ) Costaining for S100β, acetylated-tubulin and γ-tubulin in en face whole-mount preparations of the wall of the lateral ventricle of P10 mice confirmed decreased immunoreactivity of S100β and density of multiciliated ependymal cells. Scale bar, 25 μm. Full size image In order to more thoroughly analyse the integrity of the ependymal layer lining the lateral ventricles, we performed en face whole-mount staining for the simultaneous detection of S100β, acetylated-tubulin and γ-tubulin to label both cilia and basal bodies of ependymal cells ( Fig. 8c ). Whole-mount staining confirmed a reduced immunoreactivity for S100β protein, and decreased density of mature, multiciliated ependymal cells. These data together indicate a compromised organization of the ependymal cell layer in Cdh1-null newborns. p53 is required for apoptosis but not for replicative stress To obtain additional insights into the molecular pathways involved in the DNA damage and apoptotic response in Cdh1-null brain, we decided to study the effect of Cdh1 depletion in different genetic backgrounds. We first used cyclin B1 mutant mice, as cyclin B1 is a major Cdh1 substrate and cyclin B1 overexpression is known to induce apoptotic cell death in terminally differentiated neurons [25] . As complete ablation of cyclin B1 leads to embryonic lethality [29] , we analysed the survival of Fzr1 (Δ/Δ); Nes-Cre; Ccnb1 (+/−) mice harbouring a single copy of the cyclin B1-encoding gene. As represented in Fig. 9 , Fzr1 (Δ/Δ); Nes-Cre; Ccnb1 (+/−) mice display early lethality similar to Fzr1 (Δ/Δ); Nes-Cre mice with normal copies of cyclin B1, accompanied by the presence of hydrocephalus in all these mutant mice. Lack of one allele of cyclin B1 partially stabilized survival of adult animals although these differences did not reach statistical significance ( Fig. 9a ). 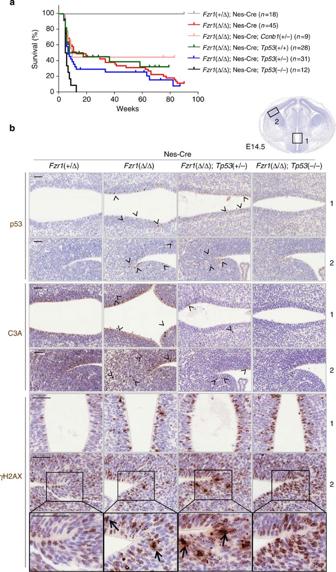Figure 9: Effect of Cdh1 ablation in different genetic backgrounds. (a) Survival curve ofFzr1(Δ/Δ); Nestin-Cre mice in aCcnb1(+/−),Tp53(+/−) orTp53(−/−) background. Only the complete ablation of p53 results in significant (P<0.001; Kaplan-Meier analysis) differences when compared withFzr1(Δ/Δ); Nestin-Cre mice. (b) Staining of p53, active caspase-3 and γH2AX inFzr1(Δ/Δ); Nestin-Cre and control cortices (1) and the ependymal layer of the third ventricle (2) in E14.5 embryos. Arrowheads indicate representative positive cells for the different stainings. Scale bar, 50 μm. Figure 9: Effect of Cdh1 ablation in different genetic backgrounds. ( a ) Survival curve of Fzr1 (Δ/Δ); Nestin-Cre mice in a Ccnb1 (+/−), Tp53 (+/−) or Tp53 (−/−) background. Only the complete ablation of p53 results in significant ( P <0.001; Kaplan-Meier analysis) differences when compared with Fzr1 (Δ/Δ); Nestin-Cre mice. ( b ) Staining of p53, active caspase-3 and γH2AX in Fzr1 (Δ/Δ); Nestin-Cre and control cortices (1) and the ependymal layer of the third ventricle (2) in E14.5 embryos. Arrowheads indicate representative positive cells for the different stainings. Scale bar, 50 μm. Full size image We next tested the effect of eliminating p53 in a Cdh1-null background. Deletion of a single allele of p53 had some effect in the survival of Cdh1-null mice, and Fzr1 (Δ/Δ); Nes-Cre; Tp53 (+/−) mice died with slightly accelerated kinetics when compared with Fzr1 (Δ/Δ); Nes-Cre; Tp53 (+/+) animals ( Fig. 9a ). Deletion of both alleles of p53 resulted in a marked acceleration of lethality within the first 10 weeks of age ( Fig. 9a ). This lethality was not because of the development of lymphomas or sarcomas typical of p53-null mice (latency ~6 months). Instead, Fzr1 (Δ/Δ); Nes-Cre; Tp53 (−/−) mice died with a more aggressive phenotype characterized by hydrocephalus and severely hypoplastic brains ( Supplementary Fig. S9 ). Importantly, no apoptosis was observed in p53-deficient embryos ( Fig. 9b ) suggesting that this protein is essential for cell death caused by Cdh1 loss. Instead, these double-mutant brains displayed an increased accumulation of cells positive for the γH2AX signal in the embryonic cortex ( Fig. 9b ). These defects were already evident during embryogenesis ( Supplementary Fig. S10 ) but were more marked at postnatal stages. The presence of the γH2AX signal was markedly increased at P10 all over the brain of Fzr1 (Δ/Δ); Nes-Cre; Tp53 (−/−) mice, including not only the ependymal layer but also cortical regions in which the damaged cells were rarely observed in Fzr1 (Δ/Δ); Nes-Cre; Tp53 (+/+) animals (4.1% in Fzr1 (Δ/Δ); Nes-Cre; Tp53 (−/−) brains versus 0.4% in Fzr1 (Δ/Δ); Nes-Cre; Tp53 (+/+) brains; Fig. 10a,b ). Damaged cells included not only Sox2- and Sox9-progenitor cells in the subventricular zone of these brains but also postmitotic neurons characterized by the cytoplasmic βIII-tubulin staining ( Fig. 10b ). Similarly, lack of p53 did not rescue the accumulation of Ki67 ( Supplementary Fig. S11 ) or G2-like pH3-positive cells ( Supplementary Fig. S12 ) but rather resulted in an accumulation of these damaged cells in the brains of Cdh1-null mice. Despite the presence of these additional damaged cells, lack of p53 did not rescue the reduced thickness of the cortex of Cdh1-deficient brains ( Supplementary Figs S11, S12 ). Indeed, double Cdh1; p53 mutant brains presented severe malformations and massive haemorrhages ( Supplementary Fig. S9 ). All together, these results suggest that p53 is not involved in the generation of replicative stress in the absence of Cdh1, but it is critical for preventing developmental defects caused by the presence of damaged, non-functional Cdh1-null cells. 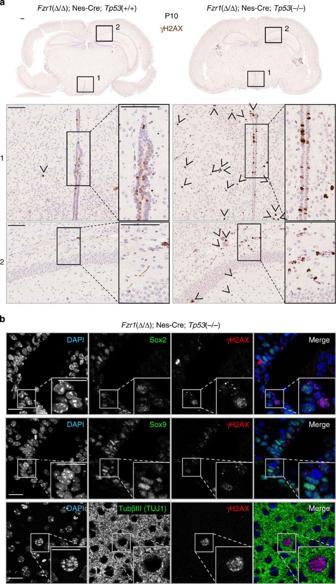Figure 10: Persistence of damaged neurons after birth in double Cdh1-p53 mutant brains. (a) Immunohistochemical analysis of phosphorylation of H2AX (γH2AX) in P10 brain sections ofFzr1(Δ/Δ); Nestin-Cre;Tp53(+/+) andFzr1(Δ/Δ); Nestin-Cre;Tp53(−/−) mice. The presence of DNA damage in the ventricles (1) and the cortex (2) is indicated by the γH2AX signal (arrowheads). (b) Immunofluorescence analysis of γH2AX, Sox2, Sox9 and neuron-specific class III beta-tubulin (βIII-Tub) showing the presence of damage in cortical postmitotic neurons ofFzr1(Δ/Δ); Nestin-Cre;p53(−/−) mutant mice. Scale bar, 100 μm (a) and 20 μm (b). Figure 10: Persistence of damaged neurons after birth in double Cdh1-p53 mutant brains. ( a ) Immunohistochemical analysis of phosphorylation of H2AX (γH2AX) in P10 brain sections of Fzr1 (Δ/Δ); Nestin-Cre; Tp53 (+/+) and Fzr1 (Δ/Δ); Nestin-Cre; Tp53 (−/−) mice. The presence of DNA damage in the ventricles (1) and the cortex (2) is indicated by the γH2AX signal (arrowheads). ( b ) Immunofluorescence analysis of γH2AX, Sox2, Sox9 and neuron-specific class III beta-tubulin (βIII-Tub) showing the presence of damage in cortical postmitotic neurons of Fzr1 (Δ/Δ); Nestin-Cre;p53(−/−) mutant mice. Scale bar, 100 μm ( a ) and 20 μm ( b ). Full size image The APC/C is an essential E3-ubiquitin ligase involved in cell cycle regulation mostly during mitosis and the following G1 phase [3] . In addition, this complex is involved in the control of metabolism and differentiation in various cell types [10] , [30] , [31] , [32] , [33] , and recent studies have suggested a crucial role for APC/C-Cdh1 and APC/C-Cdc20 in postmitotic neurons [5] , [12] , [13] , [14] , [15] , [16] , [34] . Whereas APC/C-Cdc20 targets for degradation a few critical mitotic regulators (A- and B-cyclins, Nek2 and securin), Cdh1 is more promiscuous and targets for degradation multiple cell cycle regulators including Cdc20 targets as well as Cdc20 itself [3] , [5] . Genetic ablation of Cdc20 results in a complete metaphase arrest in mammals confirming its essential role in the degradation of cyclin B and securin required for anaphase onset [6] , [7] . Cdh1, on the other hand, is not essential for the cell cycle although lack of Cdh1 results in early entry into the S phase and reduced proliferation rate [8] , [9] , [35] . Cdh1 has been proposed to mediate a DNA damage response to genotoxic stress [36] and proliferative defects caused by Cdh1 deficiency are p53 independent [35] , [37] . The irradiation-induced checkpoint is deficient in Cdh1-deficient bone marrow cells suggesting a role for Cdh1 in the G2 checkpoint in vivo [38] . Genetic deletion of Cdh1 in the mouse embryo results in placental defects owing to an essential role of this protein in endoreduplication [8] , [9] . Yet, the physiological consequences of eliminating Cdh1 in mitotic tissues in vivo are unclear. We have focused on the nervous system, as multiple evidences have suggested in the past a neural role for Cdh1 (refs 5 , 11 ). Cdh1 depletion in neural progenitors resulted in the upregulation of its known substrates and an initial increase in DNA replication. We and others have observed in the past that Cdh1-deficient cells display an early loading of replication complexes resulting in shorter G1 and premature entry into the S phase [8] , [37] . This phenotype is at least partially because of increased cyclin levels and reduced amounts of cell cycle inhibitors as a consequence of Skp2 accumulation ( Fig. 3 and Supplementary Fig. S4 ; see also refs 8 , 9 ). In fact, we have now demonstrated that the replicative stress and the proliferative defects induced by Cdh1 loss can be rescued by moderate inhibition of Cdks, suggesting that Cdk hyperactivation is one of the major mechanisms responsible for replicative stress in the absence of Cdh1. In the developing cortex, this is accompanied by the accumulation of p53, a G2-like arrest and apoptosis. These alterations also affected the ependymal layer originated from fetal neural progenitors likely resulting in hydrocephalus, a condition that is known to occur on compromised integrity of ependymal cells [27] , [28] , [39] . In fact, recent data suggest that increased death of neural progenitors is sufficient to induce hydrocephalus in the mouse, and that defects in these neural progenitors are crucial in the pathogenesis of neonatal hydrocephalus [40] . We therefore propose that Cdh1 deficiency results in replicative stress in vivo leading to a G2-like arrest and/or apoptosis of progenitor cells. In the brain, this results in a reduction in the number of neurons, tissue hypoplasia, perhaps related to microcephaly as shown for other cell cycle regulators [41] , and hydrocephalus. As suggested from in vitro studies with cultured cells [35] , [37] , p53 is not required for the proliferative defects caused by Cdh1 inhibition, and double Fzr1 (Δ/Δ); Nes-Cre; Tp53 (−/−) brains accumulated a significant amount of replicative stress. Consequently, ablation of p53 did not rescue developmental defects caused by Cdh1 ablation. Intriguingly, p53 deficiency strongly synergized with Cdh1 loss and double-mutant mice died within the first 10 weeks of life with severe brain hypoplasia and hydrocephalus. This phenotype correlated with lack of apoptosis in neural progenitors indicating that p53 is essential for the apoptotic cell death induced by Cdh1 loss ( Fig. 9 ). These results are in agreement with the reported requirements for p53 in the apoptotic death of neural progenitors with abnormal cell cycle progression induced by p57 Kip2 or Atr inactivation [42] , [43] . In fact, p53 loss has been shown to exacerbate the effects of DNA replication defects in several models [44] , [45] , [46] , further supporting the idea that the primary defect in Cdh1-deficient cells is related to abnormal DNA replication. This is likely to be related with the role of p53 in limiting DNA replication in the presence of damage. As proposed previously, in the absence of p53, initiation of DNA replication continues and DNA damage accumulates leading to a synthetic lethal interaction between replicative stress and p53 loss [44] , [46] . All together, these data suggest a major function for Cdh1 in protecting neural progenitors against unrestrained entry into the cell cycle, genomic damage and cell death. Whereas replicative stress in the absence of Cdh1 is p53 independent, p53 plays a major role in preventing developmental defects by eliminating these damaged cells from the tissue. The requirements for the APC/C during the cell cycle have promoted different studies to evaluate the relevance of this complex as a cancer target [20] . The pioneer suggestion that targeting mitotic exit is a relevant therapeutic strategy [21] has been confirmed using Cdc20-deficient mice [6] , and the first APC/C inhibitor is currently under preclinical studies [47] , [48] . Elimination of APC/C-Cdc20 activity results in metaphase arrest owing to the lack of degradation of cyclin B1, and this strategy is more efficient in killing cells than current microtubule poisons such as taxanes [6] , [21] . These therapeutic approaches are directed against APC/C-Cdc20 activity, and the concomitant inhibition of Cdh1 has been considered as a putative undesired effect owing to the proliferative potential of overexpressed Cdh1 substrates (cyclins, aurora or Plk1 kinases and so on). Contrary to these expectations, our genetic data suggest that ablation of Cdh1 results in replicative stress in vivo and a general antiproliferative response that is not p53-dependent. As Fzr1 (−/Δ); Sox2-Cre displayed defects in the development of multiple organs ( Supplementary Fig. S3 ), the antiproliferative effect caused by Cdh1 ablation is likely common to many other tissues. Thus, putative APC/C inhibitors are unlikely to generate proliferative responses even in the case of unspecific inhibition of Cdh1 and with independence of the p53 status of tumour cells. Generation and characterization of mutant mice All animals were maintained in a mixed 129/Sv (25%) × CD1 (25%) × C57BL/6J (50%) background. Mice were housed in the pathogen-free animal facility of the Centro Nacional de Investigaciones Oncológicas (Madrid, Spain) following the animal care standards of the institution. These animals were observed on a daily basis and sick mice were killed humanely in accordance with the Guidelines for Humane End Points for Animals used in biomedical research. All animal protocols were approved by the ISCIII committee (Madrid, Spain) for animal care and research. In the mouse, Cdh1 is encoded by the Fzr1 gene. Fzr1 (lox) mice [8] were used to conditionally deplete Cdh1 on Cre expression, using Tg.Sox2-Cre mice, that express Cre in embryonic but not in extra-embryonic tissues [49] or Tg.Nestin-Cre mice that express this recombinase in the developing nervous system (The Jackson Laboratory: strain name: B6.Cg-Tg(Nes-cre)1Kln/J; stock number: 003771 (ref. 22 ). Conditional expression of Cre results in the Fzr1 (Δ) allele, whereas Fzr1 (−) refers to the null allele after germline transmission. These Cdh1-deficient mice were crossed to mice heterozygous for a null mutation in the Cyclin B1 locus [29] or deficient in the tumour suppressor p53 [50] .The LSL-YFP allele contains a reporter YFP that is only expressed after recombination of the LoxP sites by the Cre recombinase [51] . For histological observation, dissected organs or E12.5–E18.5 embryos were fixed in 10%-buffered formalin (Sigma) and embedded in paraffin wax. Sections of 5 μm thickness were stained with hematoxylin and eosin. Additional immunohistochemical examination of the tissues and embryos analysed were performed using specific antibodies ( Supplementary Table S1 ). Animals underwent the object-recognition test following a protocol described previously [52] with minor modifications [8] . Briefly, seven Fzr1(Δ/Δ); Nestin-Cre and nine control Fzr1(+/Δ); Nestin-Cre adult (13–25-week-old) mice were placed in a plastic box with opaque walls. The two similar objects (objects X and Y) were plastic parallelepipeds and the dissimilar object (object Z) was a plastic bottle. Mice were first exposed to the cage and to objects X and Y. After a familiarization period, each mouse was released in the experimental cage with objects X and Z. The objects and the cage were wiped with 70% ethanol after each exposure to eliminate odour cues. The total time of recognition activity was scored manually using a stopwatch and recorded. Molecular imaging Computerized axial tomography scanning was performed on anesthetized mice (1–3% of Isoflurane (Isoba Vet)) using the eXplore ista PET-CT (GE Healthcare) with the following parameters: 200 μA, 35 kV, 160 μ, 16 shots y 360 projections. MMWKS (GE Healthcare) and MicroView software were used to analyse the images. Nuclear magnetic resonance was performed using a 4.7-tesla Biospec 47/40 (Bruker). Images of transverse relaxation time T2 were taken. Isolation and culture of neural progenitors Mouse cerebral cortices from different embryo stages (E12.5–E17.5) were dissected and gently dissociated manually, as described previously [53] . Single dissociated cortical cells were cultured in uncoated 6-well plates for 7 days in a serum-free medium containing Dulbecco's modified Eagle medium with high glucose, sodium pyruvate, glutamine, N2, B27 (all from Gibco), 2 mM N -acetyl-cysteine (Sigma) and 20 ng ml −1 each of FGF2 (Invitrogen) and EGF (Gibco) and maintained at 35 °C in 6% CO2. For subcloning, neurospheres were collected and gently dissociated using papain (Worthington) for 30 min at 37 °C with gentle agitation. Immunofluorescence and biochemical analysis EdU (10 μM) was added to neurospheres after 3–4 days of growth in vitro . After 1 h they were attached to matrigel-coated coverslips (BD Biosciences), fixed with 4% paraformaldehyde (Polysciences) for 15–20 min at room temperature (RT) and incubated with phosphate-buffered saline-Triton 0.5% for permeabilization. Neurospheres were then incubated with EdU Click-iT cocktail (Invitrogen), blocked with 3% bovine serum albumin and incubated with primary antibodies ( Supplementary Table S1 ) for 1–2 h at RT. The matching secondary antibodies (Alexa fluor 488, 594 or 647; dilution 1:500) were from Molecular Probes (Invitrogen; Catalogue numbers: A21441, A11001, A11012, A11005, A21443, A21463). Images were obtained using a laser scanning confocal microscope TCS-SP5 (AOBS) Leica. For high-throughput microscopy (HTM), neural progenitors were treated for 8 h with Roscovitine or nucleosides and EdU was added during the last 30 min. Then, they were attached to μCLEAR bottom 96-well plates (Greiner Bio-One) after disaggregation. Images were automatically acquired from each well by an Opera High-Content Screening System (Perkin Elmer). A × 20 magnification lens was used and pictures were taken at non-saturating conditions. Images were segmented using the 4′,6-diamidino-2-phenylindole (DAPI) staining to generate masks matching cell nuclei from which the γH2AX mean signal was calculated. Tissues for immunofluorescence were fixed in 10% buffered formalin (Sigma) and embedded in paraffin wax or frozen in Tissue-Tek OCT compound (Sakura). Tissue sections were blocked with 3% bovine serum albumin and incubated with primary antibodies ( Supplementary Table S1 ) for 1–2 h at RT. Secondary antibodies (Alexa 488, 594 or 647) from Molecular Probes (Invitrogen) were used and images were obtained using a laser scanning confocal microscope TCS-SP5 (AOBS) Leica. For SEZ whole-mounts, we used protocols established previously [54] . Briefly, brains from p10 newborns were extracted and the wall of the lateral ventricles was dissected and fixed in 4% paraformaldehyde – 0.1% Triton X100. Incubation with primary antibodies ( Supplementary Table S1 ) was performed for 48 h in 10% calf serum – Triton 0.1% in phosphate-buffered saline blocking buffer before incubation with appropriate secondary antibodies. Tissue was mounted using Fluormount-G (Southern Biotech). For western blotting, neurospheres were harvested after 7–9 days in vitro , lysed in RIPA buffer and 50 μg of total protein was separated by SDS–PAGE, transferred to nitrocellulose membranes (Bio-Rad) and probed with different antibodies ( Supplementary Table S1 ). The secondary antibodies (dilution 1:20000) were HRP-conjugated antibodies (DAKO; Catalogue numbers: P0447, P0448) and the western blots were developed using the ECL system (PerkinElmer). Full-blot scans of these detections are represented in Supplementary Fig. S13 . Statistical analysis All cellular experiments were repeated at least three times and analysed statistically. All data from mice are obtained at least from three different animals. Statistical analysis was performed using Student’s t- , chi-square or log-rank tests (GraphPad Prism 5). All data are shown as mean±s.d. or mean±s.e.m. ( Fig. 5 and Supplementary Fig. S7 ); probabilities of P <0.05 were considered significant. How to cite this article: Eguren, M. et al. The APC/C cofactor Cdh1 prevents replicative stress and p53-dependent cell death in neural progenitors. Nat. Commun. 4:2880 doi: 10.1038/ncomms3880 (2013).